Ruthenium-catalysed alkoxycarbonylation of alkenes with carbon dioxide Alkene carbonylations represent a major technology for the production of value-added bulk and fine chemicals. Nowadays, all industrial carbonylation processes make use of highly toxic and flammable carbon monoxide. Here we show the application of abundantly available carbon dioxide as C1 building block for the alkoxycarbonylations of industrially important olefins in the presence of a convenient and inexpensive ruthenium catalyst system. In our system, carbon dioxide works much better than the traditional combination of carbon monoxide and alcohols. The unprecedented in situ formation of carbon monoxide from carbon dioxide and alcohols permits an efficient synthesis of carboxylic acid esters, which can be used as detergents and polymer-building blocks. Notably, this transformation allows the catalytic formation of C–C bonds with carbon dioxide as C1 source and avoids the use of sensitive and/or expensive reducing agents (for example, Grignard reagents, diethylzinc or triethylaluminum). The functionalization of lower aliphatic alkenes constitutes an important basis of today’s chemical industry. Apart from polymerization and oxidation [1] , [2] , carbonylation reactions using carbon monoxide represent a major technology for the production of value-added bulk and fine chemicals from olefins [3] . In addition to industrial hydroformylation processes that provide aldehydes [4] , [5] , [6] , [7] , the alkoxycarbonylation of alkenes constitutes a straightforward approach to carboxylic acid esters [8] . On an industrial scale, the resulting aliphatic esters are mainly used for the production of detergents and polymer-building blocks. For example, the current state-of-the-art commercial process for methyl methacrylate polymers is based on the palladium-catalysed methoxycarbonylation reaction of ethylene ( Fig. 1a ) [9] . In this reaction, the catalytically active palladium(II)-hydride species is generated with the assistance of a Brønsted acid co-catalyst [10] , [11] . 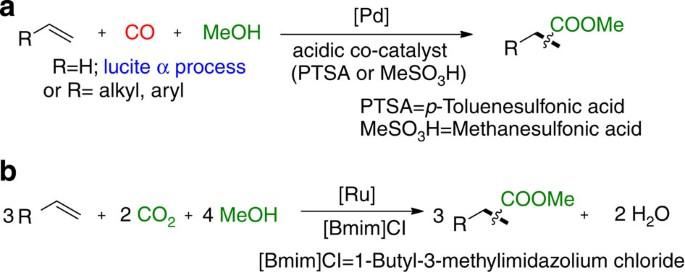Figure 1: Catalytic carbonylation of alkenes. (a) Palladium-catalysed methoxycarbonylation of alkenes with carbon monoxide and methanol to produce esters in the presence of acid co-catalyst. (b) This work: ruthenium-catalysed methoxycarbonylation of alkenes with carbon dioxide and methanol. Figure 1: Catalytic carbonylation of alkenes. ( a ) Palladium-catalysed methoxycarbonylation of alkenes with carbon monoxide and methanol to produce esters in the presence of acid co-catalyst. ( b ) This work: ruthenium-catalysed methoxycarbonylation of alkenes with carbon dioxide and methanol. Full size image Generally, all these carbonylation processes make use of toxic and flammable carbon monoxide, which is also difficult to transport on a bulk scale. More than 110,000 people protested against a pipeline for CO transport by Bayer AG in Germany. The company had to stop the installation because of this public protest; see: http://www.stopp-co-pipeline.de/ . Hence, performing carbonylations without carbon monoxide is highly desired and would further advance this area [12] . So far, all used carbon monoxide surrogates have significant drawbacks with respect to atom efficiency and/or price. For example, aldehydes [13] and higher alcohols like cinnamyl alcohol [14] or polyols [15] were used as carbon monoxide source especially in hydroformylation and Pauson–Khand-type reactions. For alkoxycarbonylation reactions, formates are known to be a CO substitute [16] . Apart from above-mentioned CO sources, stoichiometric amounts of metal carbonyls such as Mo(CO) 6 and W(CO) 6 are also applied to deliver carbon monoxide [17] . In contrast to all these protocols, the use of abundant CO 2 is desirable. However, because of its thermodynamic and kinetic stability [18] , [19] , [20] , [21] , the catalytic C–C bond formation between carbon dioxide and olefins constitutes one of the most challenging tasks for organometallic chemistry. So far, the reported carboxylation of alkenes with carbon dioxide proceeds only in the presence of (over)stoichiometric amounts of strong or expensive reductants like Et 2 Zn and silanes [22] , [23] , [24] . Obviously, such reactions are restricted because of the sensitivity and price of the reagents as well as the waste generated. In contrast, herein we describe the use of carbon dioxide as C1 source in the alkoxycarbonylation reaction of industrially important alkenes ( Fig. 1b ) and avoid the use of sensitive and/or expensive reducing agents (for example, Grignard reagents, Et 2 Zn or Et 3 Al). Furthermore, compared with the present state-of-the-art palladium-catalysed alkoxycarbonylation, advantageously in our protocol less expensive triruthenium dodecacarbonyl is applied as a convenient and stable catalyst without the usage of sensitive or acidic reagents. Effect of reaction parameters In addition to traditional carbonylation catalysts, recently ruthenium complexes demonstrated their potential in hydroformylation [25] , [26] and hydroaminomethylation reactions using CO [27] . On the basis of our expertise in this area, we became interested to use carbon dioxide as CO surrogate for such reactions. The initial experiments were carried out in high-pressure Parr reactors with 1-octene 1a in the presence of 0.5 mol% Ru 3 (CO) 12 under 40 bar carbon dioxide at 160 °C using methanol and N -methyl-2-pyrrolidone as solvent ( Supplementary Table 1 ). To our surprise, methoxycarbonylation products 2a and octane 3a were obtained in 11 and 40% yield, respectively, without any hydrogen or additional reducing agents present. Besides, significant amounts of internal octenes 4a were formed. This latter reaction is explained by the formation of ruthenium–hydride complexes, which constitute well-known alkene isomerization catalysts [28] , [29] . To favour the unusual carbonylation process, substoichiometric amounts of LiCl (0.25 equiv. to 1-octene) were added to the reaction, which are known to suppress alkene hydrogenation in the ruthenium-catalysed hydroformylation [25] , [30] , [31] . Indeed, the yield of 2a was improved to 31% ( Supplementary Table 1 , entry 2). Next, we investigated the role of additives, catalyst loading, temperature as well as solvent effects ( Supplementary Tables 1–6 ). To our delight, the corresponding methyl esters were obtained in excellent yield (>90%) using methanol as the solvent in the presence of ionic liquid as additive at 160 °C ( Fig. 2 ). Notably, good yields of the products were still achieved at lower reaction temperature (145 °C, 81% yield; Supplementary Table 1 , entry 10). 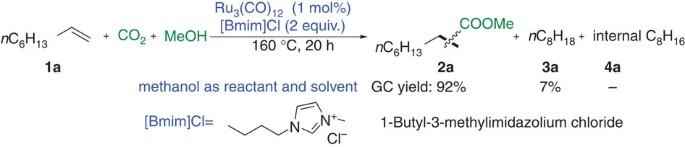Figure 2:Methoxycarbonylation of 1-octene with carbon dioxide and methanol. 1-octene 10 mmol, [Bmim]Cl 20 mmol, Ru3(CO)121.0 mol%, CO240 bar, methanol 20 ml, 160 °C, 20 h. Figure 2: Methoxycarbonylation of 1-octene with carbon dioxide and methanol . 1-octene 10 mmol, [Bmim]Cl 20 mmol, Ru 3 (CO) 12 1.0 mol%, CO 2 40 bar, methanol 20 ml, 160 °C, 20 h. Full size image Substrate scope Encouraged by these results, we studied the reactivity of different alkenes and various alcohols with carbon dioxide ( Table 1 ). Apart from methanol, 1-octene reacted well with ethanol and benzyl alcohol to produce the corresponding carboxylic acid esters in high yields (84–92%; entries 1–3). For lower terminal aliphatic alkenes, 95% of esters 5a and 6a were obtained (entries 4 and 5). In all these examples, a mixture of the branched and linear ester was formed. Looking at the kinetic profile of the benchmark reaction ( Supplementary Fig. 1 ) revealed fast conversion of 1a into 2-octene. Then, the esters 2a were produced at a lower rate along with the appearance of octane 3a and other internal octenes 4a . Thus, reactions of internal alkenes, like 2-octene, with different alcohols gave almost the same yields and selectivities compared with 1-octene (entries 6–8). In case of 1,7-octadiene, product 2a was produced with one double bond being reduced (entry 9). 3,3-Dimethylbut-1-ene gave highly selectively the corresponding terminal ester in very good yield (entries 10 and 11). Applying cyclohexene as the starting material, the generality of the process with more functionalized alcohols was studied (entries 12–23). Not only primary alcohols but also secondary alcohols reacted smoothly in moderate to excellent yields, although a longer reaction time was needed for secondary alcohols. Functionalized alcohols with halide and ether groups were well tolerated too (entries 20–23). Other cyclic olefins, for example, cyclopentene (entries 24 and 25), cis -cyclooctene (entry 26) as well as norbornene (entries 27 and 28) led to esters in 53–91% yield. Furthermore, different aromatic olefins and allyl benzene reacted with methanol or ethanol to afford a series of araliphatic esters in good yields as well (entries 29–35). Finally, methyl propionate, a bulk-scale intermediate in the manufacture of methyl methacrylate (lucite α-process), was achieved in 76% yield using ethylene as substrate (entry 36). Table 1 Alkoxycarbonylation of alkenes with carbon dioxide and alcohols*. Full size table Control experiments To gain more insight into this ruthenium-catalysed C–C bond formation [32] , [33] with carbon dioxide, a series of control experiments were performed. Initially, the reaction of carbon dioxide and methanol under catalytic conditions without any olefin present was studied ( Fig. 3a ). Interestingly, CO and H 2 were detected in the gas phase ( Supplementary Figs 3 and 4 ). At the same time, methyl formate was observed in the liquid phase. Therefore, reactions of 1-octene with these intermediates (CO, methyl formate) were conducted ( Fig. 3b,c ). As expected, ruthenium-catalysed methoxycarbonylation occurred with CO. This reaction is best achieved at low concentration of carbon monoxide ( Supplementary Table 7 ). When the carbon monoxide pressure was increased from 2 to 40 bar, the yield of the ester 2a was reduced from 70 to 31% ( Fig. 3b ). Comparing CO with CO 2 , the latter reagent is more efficient in this process (92% yield of 2a ; Fig. 3b ). We explain this unusual behaviour by the in situ formation of carbon monoxide from carbon dioxide and methanol. In addition, the control experiment with methyl formate [34] also showed esterification of the alkene 1a albeit in significantly lower yield ( Fig. 3c ). 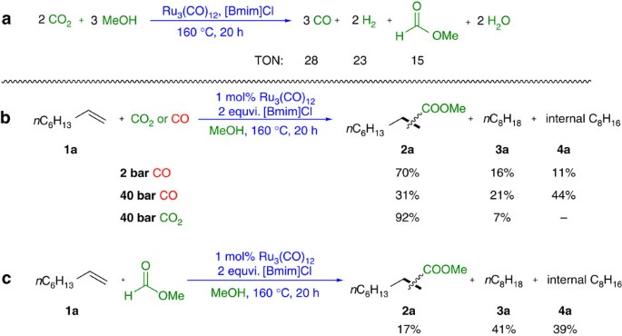Figure 3: Control experiments. (a) Analysis of standard reaction without the presence of 1-octene1a. (b) Reaction of 1-octene1awith CO (different pressures) and CO2. (c) Reaction of 1-octene1awith methyl formate. Figure 3: Control experiments. ( a ) Analysis of standard reaction without the presence of 1-octene 1a . ( b ) Reaction of 1-octene 1a with CO (different pressures) and CO 2 . ( c ) Reaction of 1-octene 1a with methyl formate. Full size image Isotope-labelling experiments To prove the origin of carbon monoxide, isotope-labelling experiments were performed. Applying 13 C-labelled carbon dioxide (12 bar) in the reactions of methanol and ethanol 82 and 86% of the carbon in the carbonyl group, respectively, were 13 C labelled ( Fig. 4a,b ). In agreement with this observation, it was revealed that only a minor amount of the carbon of the carbonyl group was 13 C labelled when 13 C-labelled methanol was applied under the same conditions ( Fig. 4c ). This result clearly demonstrated carbon dioxide as the main carbonyl source of this transformation ( Supplementary Figs 5–9 ). 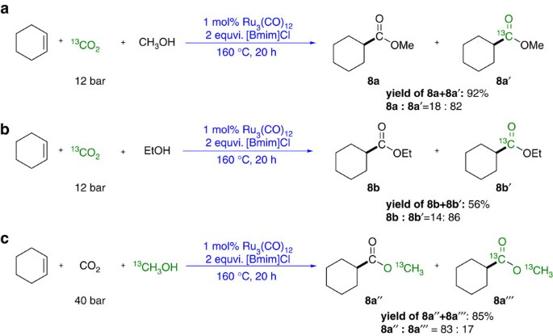Figure 4: Isotope labelling experiments. (a,b) Reactions were run in 2 mmol scale under 12 bar13CO2, other conditions were the same as inFig. 2. (c) Reaction was run in 2 mmol scale with 6 ml13CH3OH, other conditions were the same as inFig. 2. Figure 4: Isotope labelling experiments. ( a , b ) Reactions were run in 2 mmol scale under 12 bar 13 CO 2 , other conditions were the same as in Fig. 2 . ( c ) Reaction was run in 2 mmol scale with 6 ml 13 CH 3 OH, other conditions were the same as in Fig. 2 . Full size image On the basis of all these results, we suggest the following reaction pathways for alkoxycarbonylations with carbon dioxide ( Fig. 5 ): Initially, carbon dioxide is reduced by the alcohol through the so-called ‘hydrogen-borrowing’ [35] , [36] , [37] to carbon monoxide (path I) or alkyl formates (path II). Both CO and formate are detected in our reaction system and react with the alkene affording esters as discussed above. On the basis of the significantly lower yield (17%) with formate ( Fig. 3c ), we propose path I to be the major reaction pathway for this transformation. Meanwhile, the alcohol undergoes dehydrogenation to form carbonyl compounds (formaldehyde in the case of methanol; Fig. 5 , path III) [38] . Interestingly, a minor amount of the CO comes from further decarbonylation reactions as shown by the isotope-labelling experiments ( Fig. 4 ). Accordingly using p -methoxyphenyl methanol as the alcohol, small amounts of the decarbonylated product methyl phenyl ether are detected in solution [39] . 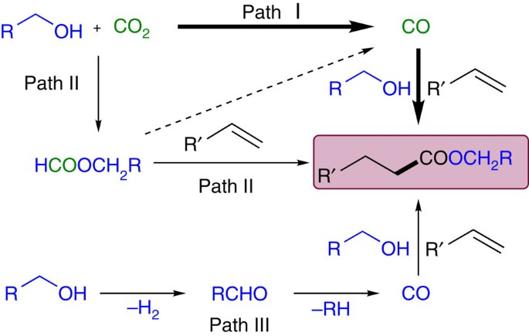Figure 5: Possible reaction pathways for the carbonylation using carbon dioxide. Path I contribute mainly to the ester production. Only minor amount of esters come from path II and III. Figure 5: Possible reaction pathways for the carbonylation using carbon dioxide. Path I contribute mainly to the ester production. Only minor amount of esters come from path II and III. Full size image While alkoxycarbonylation reactions are generally performed with homogenous catalysts, alcohol dehydrogenations are catalysed by heterogeneous catalysts. Therefore, efforts were undertaken to understand the nature of the active catalyst in this process ( Supplementary Methods ). Key experiments using 1-octene, carbon dioxide and methanol included the following: (a) the standard Hg(0) poisoning test; (b) the hot filtration test; (c) ligand poisoning and (d) control reactions with self-made ruthenium nanoparticles stabilized by ionic liquids ( Supplementary Fig. 2 ) [40] , [41] , [42] . All these tests uncovered the homogenous nature of the catalyst in this reaction system ( Supplementary Tables 8–11 ). In conclusion, we demonstrate the feasibility to use carbon dioxide and alcohols for alkoxycarbonylation processes of olefins without any additional strong reductant. A number of aliphatic olefins as well as styrenes can be transformed in high yields to industrially relevant carboxylic acid esters, for example, methyl propionate. In this process, carbon dioxide is reduced by the parent alcohol using convenient triruthenium dodecacarbonyl. The present catalyst system does not need any sensitive ligands or expensive additives. Notably, in the current ruthenium-catalysed alkoxycarbonylation process, the use of carbon dioxide and alcohols works much better than the combination of carbon monoxide and alcohols. Conceptually, it is shown that toxic carbon monoxide can be replaced by CO 2 . We estimate that this novel methodology is applicable to other carbonylation reactions too. Therefore, we anticipate that this work will contribute substantially to the development of next-generation CO 2 utilization. General analytic methods NMR spectra were recorded on Bruker Avance 300 (300 MHz) and Bruker Avance 400 (400 MHz) NMR spectrometers. Chemical shifts (p.p.m.) are given relative to solvent: references for CDCl 3 were 7.26 p.p.m. ( 1 H NMR) and 77.00 p.p.m. ( 13 C NMR). 13 C NMR spectra were acquired on a broad band-decoupled mode. Multiplets were assigned as singlet, doublet, triplet, doublet of doublet, multiplet and broad singlet. All measurements were carried out at room temperature unless otherwise stated ( Supplementary Figs 10–32 ). Electron impact mass spectra were recorded on AMD 402 mass spectrometer (70 eV). High resolution mass spectra were recorded on Agilent 6210. The data are given as mass units per charge ( m/z ). For gas chromatography (GC) analyses, HP 7890 chromatograph with a 30-m HP5 column was used. Gas-phase GC were performed on Agilent 6890N (G1530N). Isooctane is used as an internal standard for GC analysis. The products were isolated from the reaction mixture by solvent evaporation and following column chromatography on silica gel 60, 0.063–0.2 mm, 70–230 mesh (Merck) or bulb-to-bulb distillation using Büchi Glass oven B-585 wherever necessary. Linear to branched ratios were determined by GC analysis of the crude reaction mixture. Materials All commercial reagents were ordered from Acros Organics, Alfa Aesar, Aldrich or Strem. Alkenes were dried according to standard procedures. Methanol was distilled without being dried from industrial methanol. Ru 3 (CO) 12 (triruthenium dodecacarbonyl 99%) and 1-methyl-2-pyrrolidinone anhydrous (99.5%) was ordered from Aldrich and used as received. [Bmim]Cl (1-butyl-3-methylimidazolium chloride) was produced by BASF, ≥95% purity. Carbon dioxide (4.8) was received form Linde Gas. All operations were carried out by using standard high vacuum and Schlenk techniques unless otherwise noted. General procedure for the alkoxycarbonylation reaction A 100-ml autoclave was charged with Ru 3 (CO) 12 (63.9 mg, 100 μmol), [Bmim]Cl (1-butyl-3-methylimidazolium chloride, 3.48 g, 20 mmol), 20 ml alcohols and 10 mmol alkenes. Then, 40 bar of carbon dioxide was introduced before the autoclave was heated to 160 °C. After 20–36 h, the reaction was stopped by cooling down and releasing the pressure. The reaction solution was diluted with acetone and analysed by GC using isooctane as an internal standard. The products were isolated from the reaction mixture by solvent evaporation and following column chromatography on silica gel 60, 0.063–0.2 mm, 70–230 mesh (Merck) or bulb-to-bulb distillation using Büchi Glass oven B-585 wherever necessary. Methoxycarbonylation of 1-octene with CO and methanol A 100-ml autoclave was charged with Ru 3 (CO) 12 (64 mg, 100 μmol), [Bmim]Cl (1-butyl-3-methylimidazolium chloride, 3.48 g, 20 mmol), 20 ml CH 3 OH and 1.6 ml 1-octene (1.12 g, 10 mmol). Then, 2 or 40 bar of CO was introduced before the autoclave was heated to 160 °C. After 20 h, the reaction was stopped by cooling down and releasing the pressure. The reaction solution was diluted with acetone and analysed by GC using isooctane as the internal standard. The yields of corresponding products were determined as following: (1) 2 bar CO: 2a 70%, 3a 16%, 4a 11%. (2) 40 bar CO: 2a 31%, 3a 21%, 4a 44%. Methoxycarbonylation of 1-octene with methyl formate A 100-ml autoclave was charged with Ru 3 (CO) 12 (64 mg, 100 μmol), [Bmim]Cl (1-butyl-3-methylimidazolium chloride, 3.48 g, 20 mmol), 20 ml CH 3 OH and 1.6 ml 1-octene (1.12 g, 10 mmol). Methyl formate (1.2 ml) was added, and then the autoclave was heated to 160 °C. After 20 h, the reaction was stopped by cooling down and releasing the pressure (gas evolution during the reaction process). The reaction solution was diluted with acetone and analysed by GC using isooctane as the internal standard. The yields of corresponding products were determined as following: 2a 17%, 3a 41%, 4a 39%. How to cite this article: Wu, L. et al. Ruthenium-catalysed alkoxycarbonylation of alkenes with carbon dioxide. Nat. Commun. 5:3091 doi: 10.1038/ncomms4091 (2014).